Systematic analysis of somatic mutations impacting gene expression in 12 tumour types We present a novel hierarchical Bayes statistical model, xseq, to systematically quantify the impact of somatic mutations on expression profiles. We establish the theoretical framework and robust inference characteristics of the method using computational benchmarking. We then use xseq to analyse thousands of tumour data sets available through The Cancer Genome Atlas, to systematically quantify somatic mutations impacting expression profiles. We identify 30 novel cis -effect tumour suppressor gene candidates, enriched in loss-of-function mutations and biallelic inactivation. Analysis of trans -effects of mutations and copy number alterations with xseq identifies mutations in 150 genes impacting expression networks, with 89 novel predictions. We reveal two important novel characteristics of mutation impact on expression: (1) patients harbouring known driver mutations exhibit different downstream gene expression consequences; (2) expression patterns for some mutations are stable across tumour types. These results have critical implications for identification and interpretation of mutations with consequent impact on transcription in cancer. Human cancers acquire malignant properties following a stepwise accumulation of somatic genomic alterations [1] and subsequent evolutionary selection on resultant phenotypic changes. Genomic mutations (loosely classified as single-nucleotide variants (SNVs), small insertions and deletions (indels), copy number alterations and genomic rearrangements) show widespread variation in their functional impacts on gene products, biochemical pathways and phenotypic properties. Consequently, the effect of a mutation is often difficult to predict. Previous computational approaches to predict functional effects of mutations include: evolutionary conservation of the mutation sites across species, the chemical properties of amino-acid substitutions [2] and the frequency of mutations of a gene of interest relative to its expected background rate of mutations [3] . These approaches rely on interpretation of DNA sequences alone and do not consider other molecular measurements such as gene expression, methylation or proteome measurements that are co-acquired from the same tumour samples. Thus, histological or molecular context of mutations is often ignored in their interpretation. To address this deficiency, we propose that additional patterns representing functional consequences of mutations can be determined through simultaneous analysis of mutation and gene expression data. We have assessed the impact of mutations on gene expression as a means of quantifying potential phenotypic effects, and for novel cancer gene discovery. This concept is motivated by biological hypotheses predicting that some functional mutations will exhibit a ‘transcriptional shadow’, resulting from a mechanistic impact on the gene expression profile of a tumour. For example, loss-of-function mutations (nonsense mutations, frame-shifting indels, splice site mutations or homozygous copy number deletions) occurring in tumour suppressor genes such as TP53 can cause loss of expression due to nonsense-mediated messenger RNA (mRNA) decay [4] or gene dosage effects. In this context, we define a cis -effect as a genetic or epigenetic aberration that results in upregulation or downregulation of the gene itself. In contrast, some mutations can disrupt the expression of other genes in the same biochemical pathway ( trans -effects [5] ). This class of mutations tends to cast a long transcriptional shadow over many genes across the genome [5] . β-Catenin ( CTNNB1 ) mutations, which drive constitutive activation of Wnt signalling in several cancer types, are a potent example of mutational impact on gene expression. Large-scale data sets generated by international consortia provide opportunities to define the landscape of mutations impacting gene expression in thousands of tumours across the major cancer types. The Cancer Genome Atlas (TCGA) projects have generated genomic and transcriptomic data from multiple cancer types, providing a systematic characterization of somatic mutations [6] , copy number alterations [7] , oncogenic processes [8] , mutated sub-networks or pathways [9] , and genomic signature-defined tumour subtypes [10] . 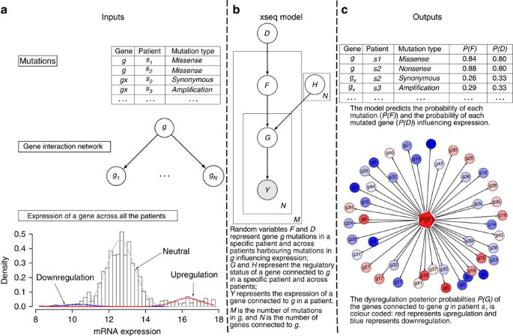Figure 1: Overview of the xseq modelling framework. (a) The inputs to the xseq model: a mutation matrix typically from next-generation sequencing, a gene interaction network and a gene expression matrix. xseq models the expression of a gene across all the patients by mixture distributions. The three mixture components represent downregulation, neutral and upregulation, respectively. (b) The graphical model representation of xseq with the plate notation. Circles represent random variables and arrows denote dependencies between variables. Boxes are plates that represent replicates. For example, the graph represents a gene mutated inMpatients (we assume that a gene is mutated only once in a patient), and the gene is connected toNgenes. (c) xseq predicts the posterior marginal probabilities of each gene (P(D)), each mutation (P(F)) influencing expression and the regulatory probabilities of the genes connected to the mutated gene in a patient (P(G)). There are few computational tools available [11] to systematically identify mutations impacting gene expression ( Supplementary Table 1 summarizes representative methods). CONEXIC [12] is a probabilistic approach to detect driver copy number regulators and their target genes. EPoC [13] derives driver copy number alterations and their target genes using differential equations to model the expression synthesis rate of a gene as a function of its copy number and the regulatory effects of other genes. MOCA [14] detects differently expressed genes in the presence of mutations in a gene, and tests the significance of the correlation (between mutation and gene differential expression). PARADIGM [15] integrates copy number and expression to identify disrupted pathways. DriverNet [16] uses a combinatorial approach and a greedy algorithm to nominate cancer driver genes. However, none of these methods can identify individual mutations that correlate with dysregulated gene networks. We present a novel statistical model, xseq, using a hierarchical Bayes approach and apply it to the analysis of thousands of tumour data sets available through TCGA, systematically examining the impact of somatic mutations on expression profiles across 12 tumour types. We demonstrate the robustness of xseq by conducting extensive computational benchmarking, and by testing xseq on an independent breast cancer data set. We identify 30 novel cis -effect tumour suppressor gene candidates, enriched in loss-of-function mutations and frequent biallelic inactivations. We identify 150 genes from trans -effect analysis impacting expression networks in the 12 cancer types, with 60 known cancer genes and 89 novel predictions. Notably, 29 of these newly predicted genes are known interacting partners of cancer driver genes. On the basis of the trans -analysis, we find two important characteristics of mutations impacting gene expression that could not be revealed with other methods: (1) a stratification of patients harbouring known driver mutations, but that exhibit different downstream gene expression consequences; (2) identification of mutations driving expression patterns that are stable across tumour types, thereby nominating important molecular targets for therapeutic intervention, transcending anatomic sites of origin. Data sets We used somatic point mutation, copy number alteration and gene expression data in 12 cancer types, from the TCGA Pan-Cancer project [17] ( Table 1 ). A total of 2,786 patients with all three types of data were included in our analyses. For trans -analysis, focal copy number homozygous deletions and amplifications (with four or more copies) predicted by GISTIC [7] , [18] were also encoded as inputs to xseq. We did not analyse the cis -effects of copy number alterations since the majority of them have cis -effects on gene expression [19] . Table 1 List of the twelve cancer types analysed. Full size table Modelling the effects of mutations on expression with xseq To address the central question of whether somatic mutations in a patient’s tumour impact gene expression, we developed a generative probabilistic model, xseq. 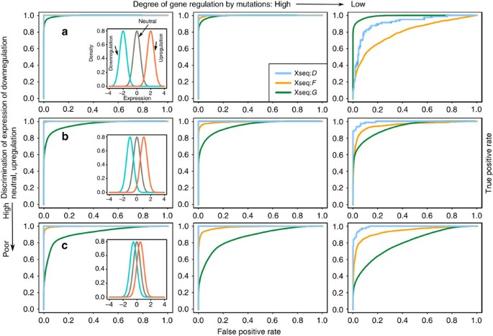Figure 2: Theoretical performance of xseq on simulated data sets. Each plot depicts a receiver operating characteristic (ROC) curve, which displays the true positive rate as a function of false-positive rate. (a) The expression of genes that are downregulated, neutral and upregulated is highly discriminative (first row), (b) moderately discriminative (second row) and (c) poorly discriminative (third row, see the enclosed figures, where cyan is downregulation, grey is neutral and red is upregulation, respectively). The ROC curves in the first column, second column and the third column were computed when the degree of dysregulation of the expression of connected genes by mutations was high, moderate and low, respectively. We present the conditional probability distributions and descriptions of the random variables of the model in Supplementary Table 2 . The model specification, assumptions and inference algorithm are fully explained in the Supplementary Methods and the Methods sections. We briefly describe them here. The xseq model is predicated on the idea that mutations with functional effects on transcription will exhibit measurable signals in mRNA transcripts biochemically related to the mutated gene—thus imposing a transcriptional shadow across part (or all) of a pathway. To infer this property, three key inputs are required for the model ( Fig. 1a ): a patient-gene matrix encoding the presence/absence of a mutation (any form of somatic genomic aberrations that can be ascribed to a gene, for example, SNVs, indels or copy number alterations); a patient-gene expression matrix encoding continuous value expression data (for example, from RNA sequencing or microarrays); and a graph structure encoding whether two genes are known to be functionally related (for example, obtained through literature, databases or co-expression data). xseq uses a precomputed ‘influence graph’ [20] as a means to incorporate prior gene–gene relationship knowledge into its modelling framework (Methods). For analysis of mutation impact in- cis , the graph reduces to the simple case where the mutated gene is only connected to itself. Given the inputs, we calculate the actual expression of the n th gene connected to mutated gene g in patient m , denoted by Y g , m , n . Figure 1: Overview of the xseq modelling framework. ( a ) The inputs to the xseq model: a mutation matrix typically from next-generation sequencing, a gene interaction network and a gene expression matrix. xseq models the expression of a gene across all the patients by mixture distributions. The three mixture components represent downregulation, neutral and upregulation, respectively. ( b ) The graphical model representation of xseq with the plate notation. Circles represent random variables and arrows denote dependencies between variables. Boxes are plates that represent replicates. For example, the graph represents a gene mutated in M patients (we assume that a gene is mutated only once in a patient), and the gene is connected to N genes. ( c ) xseq predicts the posterior marginal probabilities of each gene ( P ( D )), each mutation ( P ( F )) influencing expression and the regulatory probabilities of the genes connected to the mutated gene in a patient ( P ( G )). Full size image The output of xseq consists of: (a) the probability that a recurrently mutated gene g influences gene expression across the population of patients (denoted by P ( D g =1), Supplementary Table 2 ); and (b) the probability that an individual mutation in gene g in an individual patient m influences expression within that patient (denoted by P ( F g , m =1)). In addition to the random variables D g , F g , m and Y g , m , n , xseq also models the gene expression distribution over the patient population with gene-specific three component mixture models of Student’s t -emission densities. The three mixture components represent downregulation, neutral or upregulation, respectively ( Fig. 1a ). G g , m , n ∈ {downregulation, neutral, upregulation} denotes the status of the n th gene connected to gene g in patient m . The central assumption is that a mutation in gene g of patient m impacting gene expression (denoted by F g , m =1) more frequently co-associates with non-neutral states in its connected genes, compared with the mutations that do not impact expression. The specific direction of expression is encoded by H g , n ∈ {downregulation, upregulation} to denote the n th gene connected to gene g is upregulated or downregulated when mutations in g influence expression. (We also consider a simplified model, xseq simple without modelling the directionality of gene regulation for a specific gene, that is, without the H variable in Fig. 1b for simplicity of inference.) To represent a recurrent pattern of expression impact across multiple patients, we consider information across all patients with a mutation in gene g . This allows for borrowing of statistical strength across multiple gene expression patterns co-associating with mutations to generalize whether a mutated gene is impacting expression across the population (denoted by D g =1). ( Supplementary Fig. 1a shows a simple xseq model.) We use the Belief Propagation algorithm [21] for inference and the Expectation Maximization (EM) algorithm for parameter learning [22] ( Supplementary methods ). The inference problem is to compute the posterior probabilities P ( D g ), P ( F g , m ) and P ( G g , m , n ) given the input. The learning problem is to estimate the conditional probabilities of a variable given its parents, for example, θ F =1| D =1 —the probability of a mutation impacting expression in a specific patient given that this gene’s mutations impact expression across patients ( Fig. 1b ; Supplementary Table 2 ). For clarity of presentation, we have removed the subscripts and directly refer to D , F , G and Y . For example, we use P ( D ), P ( F ) and P ( G ) to denote the posteriors P ( D g ), P ( F g , m ) and P ( G g , m , n ), respectively. To add interpretative capacity to xseq outputs, we developed binary classifiers to determine if genes with high P ( D ) showed tumour suppressor properties P (TSG) or activating oncogenic properties P (OCG) (Methods, Modelling loss-of-function mutations and hotspot mutations). The classifiers were motivated by the pattern of distributed loss-of-function mutations across a gene for tumour suppressors (for example, TP53 ) and hotspot mutations at one or relatively few loci for oncogenes (for example, KRAS ). Computational benchmarking and validation of xseq We examined the theoretical performance of xseq via simulation and permutation analyses. To investigate the performance of xseq under different noise levels, we simulated data ( Supplementary Fig. 2 ; Supplementary Methods ) from 9 hyperparameter sets, and 10 independent realizations of data for each hyperparameter set. Overall, xseq had high sensitivity and specificity in recovering the latent variables, for example, even for the most challenging data we simulated, xseq achieved mean area under the curves of 0.99 and 0.94 for D and F , respectively ( Fig. 2 ). xseq performance was improved when given the true values for H ( Supplementary Fig. 3 ). xseq simple also performed well, but with inferior performance relative to xseq ( Supplementary Figs 4–5 ). We performed a simulation analysis of the cis -effects of somatic mutations, and found that the results were similar to those obtained from trans -simulations ( Supplementary Fig. 6 ). We also permuted the TCGA acute myeloid leukaemia ( Table 1 ) data set [23] for testing. The false discovery rates (FDRs) for D and F were 0.002 and 0.02, respectively ( Fig. 3 ; Methods). Figure 2: Theoretical performance of xseq on simulated data sets. Each plot depicts a receiver operating characteristic (ROC) curve, which displays the true positive rate as a function of false-positive rate. ( a ) The expression of genes that are downregulated, neutral and upregulated is highly discriminative (first row), ( b ) moderately discriminative (second row) and ( c ) poorly discriminative (third row, see the enclosed figures, where cyan is downregulation, grey is neutral and red is upregulation, respectively). The ROC curves in the first column, second column and the third column were computed when the degree of dysregulation of the expression of connected genes by mutations was high, moderate and low, respectively. 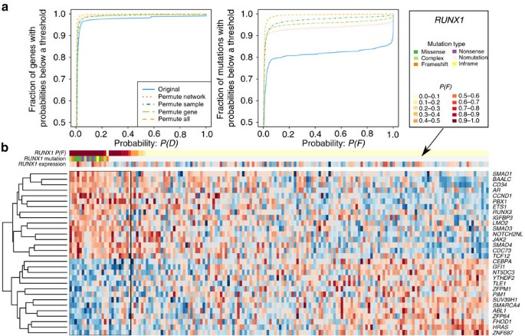Figure 3: Permutation analysis of the TCGA acute myeloid leukaemia data sets. (a) Left panel shows the empirical distribution functions ofP(D), and the right panel shows the empirical distribution functions ofP(F) estimated from different permuted data sets. (b) Heatmap shows the expression of genes connected toRUNX1: red represents high expression and blue represents low expression. Here columns represent patients and rows represent genes. For the patients withoutRUNX1mutations, we ‘assume’ the mutations still exist and estimate the probabilities of individual mutationsP(F). The mutation type ‘complex’ of a gene in a patient represents the gene harbouring multiple types of mutations in the patient. Full size image Figure 3: Permutation analysis of the TCGA acute myeloid leukaemia data sets. ( a ) Left panel shows the empirical distribution functions of P ( D ), and the right panel shows the empirical distribution functions of P ( F ) estimated from different permuted data sets. ( b ) Heatmap shows the expression of genes connected to RUNX1 : red represents high expression and blue represents low expression. Here columns represent patients and rows represent genes. For the patients without RUNX1 mutations, we ‘assume’ the mutations still exist and estimate the probabilities of individual mutations P ( F ). The mutation type ‘complex’ of a gene in a patient represents the gene harbouring multiple types of mutations in the patient. Full size image We executed a cross-validation analysis by splitting each TCGA data set into approximately equally sized discovery and validation data sets. We trained a model on the discovery data set, and used the trained model to predict the validation data set, with 10 repeats for each tumour type. We defined the validation rate as the proportion of high-probability predicted genes ( P ( D )≥0.8, see next section on picking the threshold) in the training data also predicted to have high probabilities in the validation data. For bona fide cancer genes ( Supplementary Data 1 ; Methods), the median validation rate was 0.625 across all the 12 tumour types ( Supplementary Fig. 7 ; Supplementary Table 3 ). For all of the predictions from the discovery data, the median validation rate was 0.492. The validation rate is sensitive to the number of patients (for example, the median validation rate for the predicted bona fide cancer genes in colon adenocarcinoma and breast invasive carcinoma (BRCA) was 0 and 0.73, respectively). Restricting analysis to genes with at least five mutations in both the discovery and validation data sets, median validation rates for the bona fide cancer genes and all the predicted genes increased to 0.68 and 0.63, respectively ( Supplementary Fig. 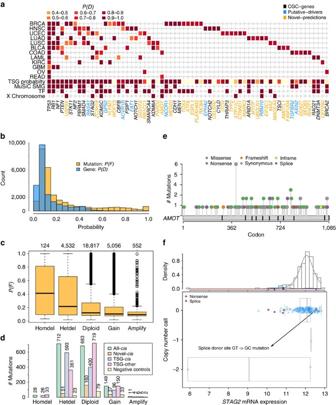Figure 4: The 65 genes harboured loss-of-function mutations with strongcis-effects on the expression of these genes. (a) The predictedcis-effect loss-of-function mutations across 12 tumour types (P(D)≥0.8 in at least one tumour type). (b) The histograms of posterior marginals of mutations and genes across tumour types. (c) The posterior marginals of mutations separated based on copy number status. (d) The loss-of-function mutations in the 65cis-effect genes (all-cis), 30 novel predictions (novelcis), 23cis-effect tumour suppressor genes (TSG-cis), 108 non-cis-effect TSGs (TSG-other) and 30 negative control genes (negative controls) segregated based on copy number status. (e) A ‘novel’ tumour suppressor geneAMOTis not significantly mutated based on frequency-based methods, butAMOTis enriched in loss-of-function mutations (tumour suppressor gene probabilityP(TSG)=0.92). (f) The loss-of-function mutations inSTAG2typically correlate with lower expression, except for a splice donor site mutation GT→GC mutation (both GT and GC are used by the splicing machinery). MuSiC SMG, significantly mutated genes predicted by MuSiC; TF, transcription factor; TSG probability, tumour suppressor gene probability. 8 ; Supplementary Table 4 ). To examine how the model would translate to independently generated data, we used the METABRIC data [5] to validate the predicted copy number alterations from TCGA in breast cancer. METABRIC copy number alterations [24] were generated with Affymetrix SNP6.0; however, gene expression was generated using Illumina microarrays. We applied the xseq model trained on the TCGA breast cancer data to analyse the METABRIC breast cancer data. 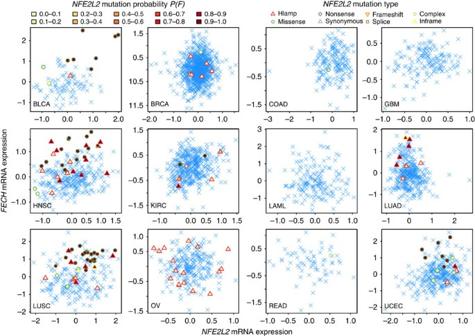Figure 5:NFE2L2mutations andFECHupregulation. NFE2L2mutations were predicted to correlate withFECHexpression upregulation in five types of cancer: BLCA, HNSC, LUAD, LUSC and UCEC. Each dot in the scatterplots represents the expression ofNFE2L2andFECHin a patient. A blue cross ‘ × ’ means the patient does not haveNFE2L2mutations. Other types of symbols represent different kinds of mutations (Hlamp, copy number amplifications). The filled colours encode the estimated mutation probabilityP(F) fromtrans-analysis (bothFECHexpression and the expression of otherNFE2L2interaction partners determineP(F)). HNSC, head and neck squamous cell carcinoma; LUAD, lung adenocarcinoma. This analysis generated 14 genes with high probability ( P ( D )≥0.8), representing a strict subset of the 42 genes predicted in the TCGA breast cancer data ( Supplementary Table 5 ; Supplementary Figs 9–10 ). Finally, we quantitatively benchmarked xseq against CONEXIC [12] and xseq simple ( Supplementary Methods ). 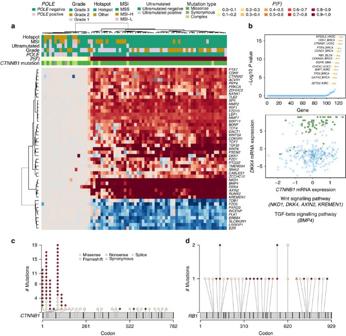Figure 6: Patients harbouring the same gene mutations but with variations intrans-associated gene expression. (a) In UCEC,CTNNB1mutations correlated with the upregulation of a set of genes, and downregulation of another set of genes. The most extreme upregulated genes includedBMP4(in TGF-β signalling pathway),NKD1,AXIN2,DKK4andKREMEN1(in Wnt signalling pathway). The downregulated genes included Wnt signalling pathway geneFZD5. Here red colour in the heatmap represents gene upregulation and blue colour represents gene downregulation. (b) The smallest unimodality dip-testPvalues ofP(F) of the 127 significantly mutated genes across tumour types. (c) The mutation sites, mutation types andP(F) (filled colours) ofCTNNB1mutations (d) andRB1mutations in UCEC. MSI, microsatellite instability; MSS microsatellite stable; MSI-H, MSI-high; MSI-L, MSI-low; TGF-β, transforming growth factor-beta. We found that xseq was more specific but potentially less sensitive than CONEXIC in predicting copy number alterations influencing expression ( Supplementary Table 6 ). xseq increased sensitivity without loss of specificity of results relative to xseq simple ( Supplementary Table 7 ; Supplementary Figs 11–12 ). Cis -effect loss-of-function mutations across the TCGA data We began analysis of the TCGA data by focusing on the cis -effect impacts of loss-of-function mutations (frameshift, nonsense and splice site mutations) on gene expression, yielding 65 genes across the 12 data sets with P ( D )≥0.8 ( Fig. 4a ; Supplementary Data 2 ). (We chose the threshold of 0.8 for P ( D ) to balance prediction of novel genes with introduction of false positives, see Supplementary Fig. 13 . Changes to the results with thresholds in the range 0.75 to 0.85 were minor.) To place these predictions in the context of known cancer genes, we compiled a list of 603 bona fide cancer genes (Methods) from the Cancer Gene Census (CGC) database [25] ( Fig. 4a , black coloured genes), Vogelstein et al . [1] and Lawrence et al . [26] ( Fig. 4a , blue coloured genes). In total, 34/65 xseq predictions overlapped bona fide cancer genes. We compared xseq predictions with those [6] predicted by an orthogonal method, MuSiC [27] , which computes the statistical significance of the population mutation frequency of a gene above an expected background mutation rate to predict its role as a cancer gene. As MuSiC uses only mutation data, and not expression data, we used it as a benchmark to determine the effect of integrating gene expression data on cancer gene discovery. MuSiC predicted 22/65 genes as significantly mutated. Importantly, 13/43 of the xseq genes that were not predicted by MuSiC were present in the list of bona fide cancer genes, suggesting that integrating gene expression information can complement the existing mutation frequency-based methods to identify mutated cancer genes. Figure 4: The 65 genes harboured loss-of-function mutations with strong cis -effects on the expression of these genes. ( a ) The predicted cis -effect loss-of-function mutations across 12 tumour types ( P ( D )≥0.8 in at least one tumour type). ( b ) The histograms of posterior marginals of mutations and genes across tumour types. ( c ) The posterior marginals of mutations separated based on copy number status. ( d ) The loss-of-function mutations in the 65 cis -effect genes (all- cis ), 30 novel predictions (novel cis ), 23 cis -effect tumour suppressor genes (TSG- cis ), 108 non- cis -effect TSGs (TSG-other) and 30 negative control genes (negative controls) segregated based on copy number status. ( e ) A ‘novel’ tumour suppressor gene AMOT is not significantly mutated based on frequency-based methods, but AMOT is enriched in loss-of-function mutations (tumour suppressor gene probability P (TSG)=0.92). ( f ) The loss-of-function mutations in STAG2 typically correlate with lower expression, except for a splice donor site mutation GT→GC mutation (both GT and GC are used by the splicing machinery). MuSiC SMG, significantly mutated genes predicted by MuSiC; TF, transcription factor; TSG probability, tumour suppressor gene probability. Full size image We next characterized the tumour suppressor properties of the 65 xseq cis -effect predictions for consistency with known patterns of enrichment for loss-of-function mutations (Methods). We found 51/65 genes with tumour suppressor characteristics ( P (TSG)≥0.2, Supplementary Fig. 14a–b ; Supplementary Data 2 ). Results were robust to a more conservative threshold, yielding 47/65 genes with P (TSG)>=0.5 ( Supplementary Fig. 15 ). The cis -effect loss-of-function mutations were co-associated with genomic copy number (one-way analysis of variance test P value<0.001, Fig. 4c–d ), with xseq cis -effect genes enriched for coincidence with hemizygous deletion (Fisher’s exact test P value<0.001, Fig. 4c–d . The statistical test method when reporting P values is omitted from this point onwards if Fisher’s exact test is used.) Additional biological characterization of the cis-effect genes suggested strong enrichment for transcription factors, phosphoproteins and X chromosome genes. Nearly half (30/65) of the cis -effect genes encode transcription factors ( Fig. 4a ; P value<0.001), as annotated in the Checkpoint database [28] . Most of the cis -effect genes (54/65, P value<0.001) encode human phosphoproteins ( Supplementary Data 2 ), consistent with recent work predicting cancer driver genes based on enriched mutations in phosphorylation regions [29] . Finally, cis -effect genes were disproportionately found on chromosome X [30] (8/65, P value<0.01; Fig. 4a ). Taken together, these data indicate xseq cis -effect predicted genes’ properties are well aligned with known characteristics of tumour suppressor genes. For the 30 novel predictions (not in our bona fide cancer driver gene list nor significantly mutated based on MuSiC analysis), we searched for literature in support of their tumour suppressor roles in cancer. In total, we found strong connections to tumour suppressor genes for at least 17 genes ( Supplementary Discussion ). The tumour suppressor roles of several of these genes have recently been elucidated (for example, UBQLN1 (ref. 31 ) and MED23 (ref. 32 )). Notably, three genes ( AMOT , AMOTL1 and ITCH ) encode proteins in the Hippo signalling pathway, involved in restraining cell division and promoting apoptosis. We further characterized the 30 genes according to criteria presented above for all the 65 genes. Of the 30 novel predictions, 18 genes accumulated enriched loss-of-function mutations ( P (TSG)≥0.2, P value<0.001), 10 genes encode transcription factors ( P value<0.05), 21 genes ( P value<0.001) encode human phosphoproteins, three genes reside on the X chromosome ( P value<0.1). All of the novel genes were rarely mutated in the 12 studied cancer types (based on MuSiC results; Supplementary Fig. 16 ). A total of 51/252 loss-of-function mutations in these genes were in hemizygous deletion regions ( P value<0.05). As a comparison with a negative control group of genes, we used the 30 genes flagged as false-positive cancer driver genes in a recent study [3] . These genes are not significantly mutated after correction for gene length, DNA replication time and other factors in estimating the background mutation rates [3] . All 30 genes had P (TSG)<0.1. In addition, loss-of-function mutations in these genes were not enriched in hemizygous deletion regions ( P value=0.7; Fig. 4c–d ) and all 30 were predicted to have probabilities P ( D )<0.6 by the xseq model (the P ( D ) histogram is in Supplementary Fig. 17 ), suggesting that the FDR for xseq is relatively low in the TCGA data, as shown in the permutation analysis. We next estimated the proportion of known tumour suppressor genes harbouring cis -effect loss-of-function mutations. We began by enumerating a set of 131 known tumour suppressor genes from both CGC [25] and Vogelstein et al . [1] ( Supplementary Data 3 ). We found that 23/131 genes (significant enrichment of cis -effect genes, P value<0.001) were predicted to exhibit cis -expression effects indicating that loss-of-function mutations in ∼ 17.6% of tumour suppressor genes yield concomitant changes in mRNA expression levels. Trans -effect mutations across the TCGA data Application of xseq to predict mutations impacting expression in trans resulted in a total of 150 genes across the 12 cancer types ( P ( D )≥0.8; Supplementary Table 7 ; Supplementary Fig. 18a ). Sixty of the 150 (40%) genes are bona fide cancer genes. We characterized these 60 trans -effect genes with annotated roles in cancer according to biological functions and found that 30/60 genes encode transcription factors ( P value<0.001), 14/60 genes encode protein kinases ( P value<0.001) and 4/60 genes ( ATRX, BAP1, KDM5A, SETD2 , P value<0.01) are chromatin regulatory factors. Moreover, 26/60 genes encode cell cycle proteins (gene ontology term: GO:0007049). By comparison, MuSiC only predicted 35/60 of these genes ( Supplementary Data 4 ). One gene ( ACVR2A ) was predicted by both xseq and MuSiC but was not in the bona fide cancer gene list. Taken together, xseq uniquely predicted 89 novel genes through trans -impacting expression analysis ( Supplementary Data 5 ). Further investigation revealed that 29/89 of the novel predicted genes were known interacting partners of previously characterized bona fide cancer genes. The gene (protein) interactions were assessed based on the high-quality protein–protein interaction networks [33] (downloaded from the Center for Cancer Systems Biology website [34] ). As for the 60 genes above, 23/89 genes encode transcription factors ( P value<0.1), 7/89 genes encode protein kinases ( P value<0.05), 3/89 genes are chromatin regulatory factors ( P value<0.1), 18/89 genes encode proteins of the cell cycle process ( P value<0.01). Pathway analysis indicated these genes encode proteins involved in major cancer pathways such as cell proliferation, apoptotic process, mitotic cell cycle, chromatin modification, cell migration and focal adhesion ( Supplementary Data 6 ). Nineteen genes were predicted to have P (TSG) or P (OCG)≥0.2 ( Supplementary Data 5 ). The gene which harboured the largest number of high-probability mutations was KPNA2 in breast cancer ( Supplementary Fig. 19, 43 mutations with P ( F )≥0.5. As shown in Supplementary Fig. 18b–c , P ( F ) follows a bimodal distribution centred at 0 and 1. Results are similar if choosing slightly different thresholds for P ( F ).) To examine other sources of evidence of functional effects, we analysed high-probability missense mutations across all the tumour types, and computed the enrichment of phosphorylation-related SNVs (pSNVs) [29] , [35] . (We found 839 missense mutations with P ( F )≥0.5 in the genes with P ( D )≥0.8, and also overlapped the set of missense mutations analysed [35] .) Of these mutations, 620 were unique when the same amino-acid residue replacement in different patients was considered. We performed two analyses where the same amino-acid substitution missense mutations (from different patients) were considered as separate events or collapsed into the same event (unique). The Pan-Cancer data set included 241,700 (236,367 unique) missense mutations. Among them, 16,840 (16,074 unique) mutations were pSNVs. Of the high-probability SNVs, 232/839 of them were pSNVs (134/620 unique). The high-probability missense mutations were highly enriched in pSNVs in both analyses ( P value <0.001). These results provided additional data to support functional activity of the xseq predictions specifically related to impact on phosphorylation. Expression dysregulation across tumour types Certain genes are frequently mutated in multiple tumour types [6] . We asked whether these mutations across tumour types correlated with the dysregulation of the same set of genes. We focused on those genes whose mutations were predicted to influence gene expression in multiple tumour types. For each gene connected to the mutated gene g in a tumour type, we counted how many times this gene was dysregulated ( P ( G =‘upregulation’)≥0.5 or P ( G =‘downregulation’)≥0.5) in the presence of high-probability mutations ( P ( F )≥0.5). We analysed downregulation and upregulation independently using a binomial exact test to test the significance of this correlation (high-probability mutations and gene dysregulation). The binomial distribution parameters were obtained by maximum likelihood estimation from all count data. From this analysis, we found 17/20 recurrent genes had at least 1 gene upregulated or downregulated in 2 tumour types ( Supplementary Data 7 , 8 ). Mutations in RB1 correlated with the same group of gene dysregulations across several tumour types. In particular, we observed that RB1 mutations correlated with E2F family gene upregulations (for example, E2F1 ; Supplementary Data 7 ; Supplementary Fig. 20 ) in bladder urothelial carcinoma (BLCA), BRCA, glioblastoma multiforme (GBM), lung squamous cell carcinoma (LUSC), ovarian serous cystadenocarcinoma (OV) and uterine corpus endometrioid carcinoma (UCEC; Table 1 ), as well as genes encoding mini-chromosome maintenance proteins, for example, MCM5 ( Supplementary Data 7 ; Supplementary Fig. 21 ) in BRCA, GBM, lung adenocarcinoma, LUSC and OV. To confirm these correlations, for each gene connected to RB1 in the original full influence graph (Methods), in each tumour type, we compared the expression of this gene in the patients with RB1 mutations to the patients without RB1 mutations using the Limma package [36] . We then aggregated all the obtained P values from the genes connected to RB1 across tumour types, and computed the FDRs [37] . We found that E2F1 was upregulated in BLCA, BRCA, GBM, LUSC and UCEC (FDR<0.1, Supplementary Fig. 22 ). We performed a similar analysis for MCM5 and found it was upregulated in BRCA, GBM, LUSC, OV and UCEC (FDR<0.1; Supplementary Fig. 23 ). In addition, aberrations (mutations and amplifications) in the transcription factor NFE2L2 in six different tumour types (BLCA, head and neck squamous cell carcinoma, kidney renal clear cell carcinoma, lung adenocarcinoma, LUSC and UCEC) exhibited trans -effects on gene expression ( P ( D )≥0.8). Two genes, MAFG ( Supplementary Figs 24–25 ) and FECH ( Fig. 5 ; Supplementary Fig. 26 ) were significantly upregulated in five and four tumour types, respectively, in the presence of NFE2L2 aberrations (FDR<0.1; Supplementary Data 7 ). As MAFG , FECH and NFE2L2 reside on chromosome 17, 18 and 2, respectively, the correlations are not likely caused by gene dosage effects. Several other genes were also upregulated in the presence of NFE2L2 aberrations, for example, NQO1, TXNRD1, PRDX1, GSR, GPX2, GCLM, FTL, AKR1C1, TXN, SQSTM1, GSTA1, KEAP1, GSTA4, ABCC1 , and GCLC were upregulated in six to three tumour types ( Supplementary Data 7 ). The boxplots in Supplementary Fig. 27 and the scatter plots in Supplementary Fig. 28 show the correlation between NFE2L2 aberrations and its direct regulator and binding partner, KEAP1 expression upregulation. Figure 5: NFE2L2 mutations and FECH upregulation. NFE2L2 mutations were predicted to correlate with FECH expression upregulation in five types of cancer: BLCA, HNSC, LUAD, LUSC and UCEC. Each dot in the scatterplots represents the expression of NFE2L2 and FECH in a patient. A blue cross ‘ × ’ means the patient does not have NFE2L2 mutations. Other types of symbols represent different kinds of mutations (Hlamp, copy number amplifications). The filled colours encode the estimated mutation probability P ( F ) from trans -analysis (both FECH expression and the expression of other NFE2L2 interaction partners determine P ( F )). HNSC, head and neck squamous cell carcinoma; LUAD, lung adenocarcinoma. Full size image Stratifying patients harbouring the same gene mutations We investigated whether xseq probabilities P ( F ) could stratify patients harbouring mutations in the same cancer driver gene. We analysed each of the 127 genes from Kandoth et al . [6] in each tumour type for the presence of bimodal xseq P ( F ) distributions over patients harbouring mutations in the genes of interest ( Supplementary Methods ). Twenty-two commonly mutated genes exhibited bimodal distributions in at least one tumour type ( Supplementary Table 8 ; Fig. 6b ; Supplementary Fig. 29 ). This was particularly evident for CTNNB1 mutations in UCEC ( Fig. 6a ); 53/72 patients harboured high-probability CTNNB1 mutations ( P ( F )≥0.5), with all 53 patients harbouring CTNNB1 hotspot mutations (mutations hitting codons between 31 and 45). By contrast, only 9/19 patients without high xseq probability CTNNB1 mutations harboured hotspot mutations ( Fig. 6c ). In addition, 9/19 patients harboured POLE mutations, or were annotated as ‘ultramutated’ (tumours with more mutations than Q3+IQR × 4.5, where Q3 is the third quartile of mutation counts across a corresponding tumour type, and IQR is the interquartile range, as defined in syn1729383), suggesting that the CTNNB1 mutations were inconsequential passenger mutations ( Supplementary Fig. 30 , CTNNB1 P ( F ) distribution). Moreover, patients in the P ( F )≥0.5 group were significantly younger than patients with P ( F )<0.5 (mean age 57.5 versus 65.7 years old, one-sided t -test P value<0.01). Figure 6: Patients harbouring the same gene mutations but with variations in trans -associated gene expression. ( a ) In UCEC, CTNNB1 mutations correlated with the upregulation of a set of genes, and downregulation of another set of genes. The most extreme upregulated genes included BMP4 (in TGF-β signalling pathway), NKD1 , AXIN2 , DKK4 and KREMEN1 (in Wnt signalling pathway). The downregulated genes included Wnt signalling pathway gene FZD5 . Here red colour in the heatmap represents gene upregulation and blue colour represents gene downregulation. ( b ) The smallest unimodality dip-test P values of P ( F ) of the 127 significantly mutated genes across tumour types. ( c ) The mutation sites, mutation types and P ( F ) (filled colours) of CTNNB1 mutations ( d ) and RB1 mutations in UCEC. MSI, microsatellite instability; MSS microsatellite stable; MSI-H, MSI-high; MSI-L, MSI-low; TGF-β, transforming growth factor-beta. Full size image Similar results for RB1 mutations in UCEC are shown in Fig. 6d . All 11 loss-of-function mutations (in eight patients) were predicted to have high probabilities ( P ( F )≥0.5); however, only 2/13 patients that did not harbour loss-of-function mutations were predicted to accumulate high-probability mutations ( P ( F )≥0.5, Fig. 6d ). Taken together, although genes such as CTNNB1 and RB1 frequently harbour driver mutations, they still likely accumulate passenger mutations without impact on gene expression. As such, patients’ tumours with these ‘inert’ mutations do not exhibit expected pathway dysregulation. xseq is therefore capable of sub-stratifying patients into meaningful phenotypic groups, separating patients with mutations and dysregulated pathways from those patients with mutations, but normal pathway activities. TP53 mutations in UCEC also showed bimodal distributions ( Supplementary Fig. 31 ). TP53 frequently accumulates both loss-of-function mutations and missense mutations. The variation in P ( F ) cannot be explained by the types and positions of the mutations ( Supplementary Fig. 32 ). However, patients with P ( F )>=0.5 were more likely to harbour copy number hemizygous deletions (36 patients harboured co-occurring hemizygous deletions, compared with eight patients with P ( F )<0.5; only nine patients lacked copy number alterations in the group with P ( F )≥0.5 compared with 12 in the group with P ( F )<0.5, P value<0.005.) We developed a probabilistic model, xseq to quantitatively assess the association of mutations with dysregulated gene expression in 12 tumour types. Computational benchmarking and assessment of independent data sets have demonstrated the robustness of xseq. Our results have implications for the interpretation of somatic mutations in retrospective, discovery-based studies. Systematic analysis of mutation and expression landscapes from >2,700 tumours uncovered several novel patterns. We revealed 30 novel tumour suppressor candidate genes by cis -effect loss of expression analysis. These genes showed the hallmarks of tumour suppressor genes including a distribution of loss-of-function mutations, and biallelic inactivation through loss-of-function mutations and heterozygous deletions. In addition, we assessed the landscape of mutations impacting gene expression in trans across the 12 tumour types. These results implicated 89 novel genes with mutations impacting gene expression. In total, 33% of these genes had functional relationships with cancer genes in core tumourigenic processes. These genes were not nominated by mutation analysis alone, suggesting that integrated analysis of mutations and gene expression is a complementary approach towards comprehensive identification of functional mutations. Recent synthesis of mutation rates and discovery ‘saturation’ in genome-wide sequencing studies has indicated that current standard of study design has under-sampled important mutations, and that for some 50 tumour types, sequencing of >2,000 cases are needed to reach comprehensive sampling [26] . The combined cis - and trans -analyses led to the elucidation of >100 novel candidate cancer genes predicted to impact expression. Integration of gene expression data directly into analysis of mutations will therefore help to bridge the discovery gap left by DNA mutation analysis alone. Results from xseq analysis identified two important characteristics for biological interpretation of mutations. The trans -analysis revealed that the same mutated gene in different patients can exhibit distinct expression impacts. In our analysis, constitutive activation of Wnt signalling genes due to CTNNB1 mutation segregates almost exclusively with known hotspot mutations. However, several cases exhibited mutation in CTNNB1 without evidence of Wnt activation, resulting in low xseq probabilities. These cases were primarily phenotyped as hypermutators due to mismatch repair deficiency and/or POLE mutations [38] , and patients were statistically older at diagnosis. Thus, a real phenotypic distinction associates with low and high xseq P ( F ) probabilities, providing evidence for integrative analysis of mutations and expression as a route to stratifying phenotypically distinct tumours in the context of the same mutations. xseq analysis identified several genes that had consistent expression impact across tumour types. Despite distinct histologies and cell contexts of source tumours, RB1 loss-of-function mutations and NFE2L2 mutations/amplifications exhibited similar expression patterns. RB1 binds and inhibits the E2F transcription factor family. Accordingly, we observed that RB1 mutations correlated with E2F family gene upregulation across tumour types. NFE2L2 binds to its regulator KEAP1 and regulates the expression of antioxidant-related genes to protect against oxidative damage. We observed NFE2L2 mutations correlated with upregulation of KEAP1 , as well as of oxidative stress genes (for example, GCLM, GCLC, TXNRD1, GPX2 and NQO1 ). While therapeutic responses to targeted inhibitors administered against the same mutation can have variable effects due to intrinsic gene expression context (for example, BRAF inhibition in melanoma and colorectal cancer [39] ), the mutations we outlined (such as RB1 and NFE2L2 mutations) exhibit stable profiles and represent important targets for future development of broadly applicable therapeutics. An intriguing evolutionary implication arises from these mutations: phenotypic impact is selected for in multiple heterogeneous tumour microenvironments, indicating independent convergence of phenotype transcending cell context. xseq is not able to distinguish different mutations of a gene within a specific patient—a limitation, as these mutations may result in different functional impacts. Although genes are rarely mutated multiple times within a single patient, some large tumour suppressor genes (such as ARID1A ) accumulate multiple mutations, as a result of their long coding sequences. Similarly, in glioblastoma and lung cancers, EGFR is frequently mutated multiple times in single patients, often due to the emergence of clonal populations following the administration of EGFR inhibitors [40] . Examining the expression impact properties of such mutations in clonal populations would likely require advanced single-cell methods [41] . In conclusion, this work provides a route towards closing the cancer gene discovery gap in the field of cancer genome sequencing. Direct, model-based integration of mutations and co-acquired gene expression measurements from tumour samples enhances interpretation capacity of discovered mutations leading to optimal selectivity of targets for functional studies and development of novel therapeutics. A generative model of the effects of mutations on expression The xseq model specifies how the expression Y of a group of genes in a patient is influenced by the somatic mutation status of a gene g in the patient ( Fig. 1b ; Supplementary Fig. 1 ). The main question we address is whether gene g co-associates with disrupted expression to itself ( cis -method) or its connected genes as defined by an influence graph (see below). On the basis of the xseq model structure in Fig. 1b , for a mutated gene g , xseq specifies a joint distribution [42] (assuming g is mutated in M patients and g has N connected genes): where is the indicator function, and when x =TRUE, otherwise . The θ s are the parameters (conditional probabilities) of xseq ( Supplementary Table 2 ). These parameters can take different values based on the subscripts, for example, θ D can take θ D =0 and θ D =1 based on the value of D . For simplicity, we consider the case with only one mutated gene and we remove ‘ g ’ in the notations. Here we assume that a gene is just mutated once in a specific patient, that is, M equals to the number of accumulated mutations in gene g . Therefore, m is the patient (mutation) index, and n is the gene index, that is, Y m , n represents the expression of the n th gene connected to g in the m th patients harbouring mutations in g . We now explain how we execute parameter learning and inference over this joint distribution. Inference of latent variables and parameter estimation It is computationally intractable to marginalize the joint distribution in equation (1) to infer the posterior marginals P ( D ), P ( F ) and P ( G ). Instead, xseq uses the belief propagation algorithm [21] , [43] to efficiently do exact inference of these posterior marginals. Here we assume that the variable means downregulation of expression and upregulation of expression, respectively) has been estimated (estimation of H is discussed below). Then, we can convert the non-tree-structured xseq model to a tree for efficient inference ( Supplementary Methods ). The belief propagation algorithm has time and memory complexity exponential in the maximum number of parents per node (two for xseq when H is given). Detailed descriptions of the belief propagation algorithm for xseq inference can be found in Supplementary Methods . The EM algorithm [22] is used to learn the parameters ( Supplementary Table 2 ) in xseq. EM algorithm iterates between the E-step and the M-step to find a local maximum of the objective likelihood function. Below, we listed the M-step update equations, and present the detailed derivations of the formulas in Supplementary Methods . The terms P ( D | Y ), P ( F , D | Y ), P ( G , F =0 | Y ) and P ( G , F =1 | Y , H ) are computed in the E-step using the belief propagation algorithm. Fixing H is key for converting the model to a tree structure for efficient inference and learning ( Supplementary Methods ). There may be several ways to estimate H , for example, using differential expression analysis to test whether a gene is upregulated or downregulated, or directly getting this information from pathway databases. In our experiments, to systematically analyse all the data sets, for the n th gene connected to gene g , we estimate the upregulation probability by , where m is the m th patients harbouring gene g mutations, M is the total number of patients harbouring gene g mutations and y m , n is the expression of the n th gene connected to g in patient m . means downregulation, neutral and upregulation of the n th gene connected to g in patient m , respectively. The probability P ( G m , n = | y m , n ) is estimated off-line by the posterior distribution of y m , n being generated from the ‘upregulation’ component (see Conditional distributions of gene expression values). Similarly, we can estimate the downregulation probability: . Conditional distributions of gene expression values The conditional distributions p ( Y = y | G ) are modelled as Student’s t -distributions and estimated off-line. For example, the conditional distribution of gene g expression distribution is modelled as a Student’s t -distribution when gene g is downregulated: where y is the expression level of gene g , and ν are the parameters of the Student’s t -distribution. As the parameter ν increases, the Student’s t -distribution approaches a Gaussian distribution . Compared with Gaussian distributions, the Student’s t -distributions are more robust to outliers, especially when ν is small. Now, the observed gene expression distribution is a mixture of three Student’s t -distribution: where ω k is the mixture weight of mixture component k . We also use the EM algorithm to uncover the parameters of the Student’s t -distributions. Influence graph In principle, the influence graph can be any such graph encoding gene regulation. The i th vertex of the graph represents gene (protein) g i and edge w i , j represents the association strength between gene (protein) g i and g j . For analysis presented in this study, we constructed a combined functional gene association network by merging the STRING v9.1 (ref. 44 ) functional protein association network, the pathway data sets from KEGG [45] , WikiPathway [46] and BioCyc [47] , and transcription factor-targets networks. The pathways have already been integrated into the IntPath database [48] . The transcription factor-targets network [49] is downloaded through the transcription factor encyclopedia web API. The ENCODE [50] transcription factor ‘proximal’ and ‘distal’ networks are also included in the combined network (download from the website [51] ). The majority of these interactions are transcription factor-target gene interactions ( ∼ 1% between transcription factor interactions in the ‘proximal’ network [50] ). For each data set, we construct a weighted network. The weight of an interaction represents our prior confidence of the interaction. For the data sets that do not provide weights for interactions, a default weight of 0.8 is used. The STRING protein–protein interaction network is already a weighted network so we use their provided weights. To merge these networks, for a specific interaction, we take the largest weight for this interaction across different networks. We then only keep the interactions with at least median confidence (threshold of 0.4, the default threshold suggested for the STRING database). In this combined network, 17,258 genes (proteins) connect to 19,070 genes (proteins) through 898,032 interactions. This network is almost weakly connected (22 genes do not connect to rest genes). Then, for each mutated gene, we test whether the genes connected to it are differentially expressed with adjusted P value (BH method) threshold of 0.05. If there exist differentially expressed genes, we only keep these genes and set their connection weights to 1. In addition, if a gene is not differently expressed in a specific tumour type but differently expressed in other tumour types based on Fishers’ combined P value FDR≤0.05, we also set their connection weights to 1. If no differentially expressed genes exist for a given mutated gene, we use the network from the original weighted network. Code availability The model and the influence and learning algorithms have been implemented in the statistical programming language R [52] , and can be downloaded from The Comprehensive R Archive Network [53] , or from our website [54] . Permutation analysis We performed several permutations to investigate the influence of each component of xseq on the final predictions. First, we switched the patient names within the mutation matrix ( Fig. 3a , permute sample; Supplementary Figs 33–34 ). Even after permutation, some mutations were still predicted to have high probabilities P ( F ). To help explain this phenomenon, we generated an expression heatmap ( Fig. 3b ), which showed the expression of genes connected to RUNX1 . We can see that some patients without RUNX1 mutations still showed similar expression pattern to those with RUNX1 mutations. This ‘phenocopy’ [55] effect could result in some patients without mutations but high predicted probabilities P ( F ). Phenocopying may be a common event in cancer because of DNA methylation and other epigenetic alterations, and it may suggest novel treatment opportunities. For example, there is increasing evidence that treating of patients based on phenotypes (expression) instead of genotypes (DNA mutations) produces better outcomes in some types of cancer [56] . We also switched the gene names within the mutation matrix ( Fig. 3a , permute gene), and the results showed similar performance to those by switching patients. Next, we randomly drew the same number of connected genes as given by the combined network ( Fig. 3a , permute network). Because the gene regulation information is sparse and some master regulators can influence the expression of huge number of genes, the model may still predict a few mutations with high probability P ( F ) because these ‘randomly drawn’ genes might be truly regulated by the mutated genes. Finally, if both the mutation matrix and the network were shuffled, there were very few predicted high-probability mutations (dashed orange curves in Fig. 3a , permute all). We performed the same processing steps after permutations thus minimizing the possibility of introducing bias. In addition, we kept the expression matrix the same in all permutation analyses. Collecting bona fide driver genes We collected the genes from the manually curated, and widely used CGC database [25] and two major recent review papers [1] , [26] as our reference bona fide cancer driver genes. Specifically, we collected 519 genes from CGC [25] , 125 genes predicted by the ‘20/20 rule’ [1] (more details below), 66 recently discovered frequently mutated genes collected in the Supplementary Table 4 of Lawrence et al [26] and 33 genes predicted by MutSig and have strong and consistent connections to cancer [26] . In summary, these data sets include 603 unique genes in total ( Supplementary Data 1 ). The 127 significantly mutated genes predicted by the MuSiC suite [6] are not counted because we use this data set for several comparisons. Notice that in our analysis, we use the samples with expression, copy number alterations and mutations. Therefore, xseq analyzes a subset of mutations used by the MuSiC suite. Modelling loss-of-function mutations and hotspot mutations The mutation patterns of most known tumour suppressor genes, and oncogenes are highly characteristic and non-random [1] . In a recent review [1] , a ‘20/20 rule’ is used to identify driver genes: for oncogenes, at least 20% of all the mutations are required to be hotspot missense mutations or in-frame indels; for tumour suppressor genes, at least 20% of all the mutations are required to be loss-of-function mutations. Here we extend the ‘20/20 rule’ using mixture-of-binomial modelling of loss-of-function mutations and hotspot mutations. We analyse oncogenes and tumour suppressor genes separately. When predicting oncogenes, we first count the number of hotspot mutations n g ,rec (recurrent missense mutations and in-frame indels) in gene g and the total number of mutations N g in gene g . Then, we model the mutation count distribution as a mixture of two binomial distributions: one component for oncogenes and the other component for non-oncogenes: Then P (OCG) is defined as the posterior of n g ,rec in the mixture component with higher success rate, namely p 1 here. The mixture parameters ω =( ω 1 , ω 2 ) and success rates p =( p 1 , p 2 ) are estimated by the EM algorithm. Similarly, when predicting tumour suppressor genes, we first count the number of loss-of-function mutations n g ,loss in gene g , and N g . Then, we model the count distribution as a mixture of two binomial distributions: one component representing tumour suppressor genes and the other representing non-tumour suppressor genes: P (TSG) is defined as the posterior of n g ,loss in the mixture component with higher success rate ( p 1 here). Again, the mixture parameters ω and success rates p are estimated by the EM algorithm. The mixture-of-binomial approach can be considered as a generation of the ‘20/20 rule’ because of its ability to estimate the parameters from data, and to account for the total number of mutations to compute posterior probabilities of genes to be oncogenes or tumour suppressor genes. To make the estimated parameters more accurate, we also added extra genome-wide screen data from COSMIC v64 (ref. 57 ), downloaded from syn1855816, and the Pan-Cancer data downloaded from syn1710680. Supplementary Figure 14 shows the binomial mixture modelling of oncogenes and tumour suppressor genes for all the genome-wide screen somatic mutation data. We used a threshold of 0.2 for P (TSG) and P (OCG) to call genes with tumour suppressor gene properties and oncogene properties, respectively ( Supplementary Fig. 15 ). Expression information in predicting driver mutations Some mutated genes are not expressed in cancer cells, and therefore the mutations in these genes are less likely to be pathogenic. Currently, the expression information has not yet been fully explored for the identification of driver mutations [58] , and only a few methods take expression information into account to assess the background mutation rates [3] . We adopted a mixture modelling approach to predict whether a gene is ‘highly expressed’ in a tumour type. We first log 2 transform the tumour gene RNA-seq by Expectation Maximization (RSEM) abundance estimation values. To prevent taking the log 2 of 0, we remove the gene expression values if they are ⩽ before log 2 -transformation. We then compute the 90th percentile of the expression of a gene across patients in a tumour type to represent the overall expression of that gene. Here we use the 90th percentile instead of median considering the gene dosage effects of copy number deletions on expression in cancer. It is unlikely that a gene is deleted in 90% of all the analysed samples (for example, for the Pan-Cancer data sets, the mostly frequently homozygously deleted gene is CDKN2A , which is deleted in 57% of patients in GBM). If we also consider heterozygous deletions, then the most frequently deleted gene is EBF3 , which is deleted in 90% of patients in GBM. The 90th percentile expression of a gene may overestimate the expression level of the gene in the studied tumour type (since we are more concerned about losing important genes). Next, we model the 90th percentile expression of genes as a mixture of two Gaussian distributions: one component representing ‘highly expressed’ and the other component representing ‘lowly expressed’. A gene is considered to be ‘highly expressed’ if its posterior probability in the ‘highly expressed’ group is ≥0.8. In the presence of outliers (some genes are expressed at extremely high or low levels), we first remove outliers based on the boxplot rule, and then fit the data. We assign a posterior probability of 1 to the highly expressed outliers, and a posterior probability of 0 to the lowly expressed outliers. Supplementary Figure 35 shows Gaussian mixture modelling of expression across the 12 cancer types. We note parenthetically that another approach to prevent taking log 2 of 0 is to add a small number, for example, 0.5 to the RSEM abundance estimation values before log 2 transformation [59] . As we use 90th percentile of the expression of a gene across patients to represent the expression of that gene, this approach may result in many lowly expressed genes to have exactly the same expression value ( Supplementary Fig. 36a , gene expression data from acute myeloid leukaemia). Consequently, a mixture of Gaussian distributions may not fit the data well since it is rare to observe exact the same value from a continuous distribution. Despite this limitation, posterior probabilities computed from both approaches are highly correlated as can be seen from the scatter plots in Supplementary Fig. 36b (Pearson correlation coefficient of 0.984, Spearman correlation coefficient of 0.995). Compensating for the cis -effects of copy number alterations Before analysing the trans -effects of somatic mutations, we first remove the cis -effects of copy number alterations on expression; copy number alterations are common in cancer and the majority have cis -effects on expression. Numerous studies have carried out integrative analysis of copy number and gene expression data [60] , [61] , [62] , [63] . Here we use the Gaussian process (GP) regression to model the expression y i of a gene in a patient i , as a function of its copy number log2 value x i . GP regression is flexible to add extra variables such as DNA methylation data as independent variables if necessary, and can capture nonlinear relationships between copy number alterations and expression. GP regression models the joint distribution of y i as a joint Gaussian distribution. The covariance matrix is constructed based on the given copy number data, cov( x i , x j )= k ( x i , x j ), where k is the squared exponential kernel function. The hyperparameters of the kernel function are computed by optimizing the log-marginal likelihood function using scaled conjugate gradient algorithms. To remove the cis -effects of copy number alterations, we subtract the regression values from the original expression values to get the residuals that are considered to be regulated by trans -effect mutations. Supplementary Figure 37 shows the scatter plots of copy number alteration and expression values for PTEN across the 12 cancer types. The GP regression lines and the 95% confidence intervals of the regression lines are overlaid on the scatter plots. Supplementary Figure 38 shows the scatter plots of PTEN expression across cancer types after removing the cis -effects of copy number alterations on expression. How to cite this article: Ding, J. et al . Systematic analysis of somatic mutations impacting gene expression in 12 tumour types. Nat. Commun . 6:8554 doi: 10.1038/ncomms9554 (2015).